Colour-tunable fluorescent multiblock micelles Emerging strategies based on the self-assembly of block copolymers have recently enabled the bottom-up fabrication of nanostructured materials with spatially distinct functional regions. Concurrently, a drive for further miniaturization in applications such as optics, electronics and diagnostic technology has led to intense interest in nanomaterials with well-defined patterns of emission colour. Using a series of fluorescent block copolymers and the crystallization-driven living self-assembly approach, we herein describe the synthesis of multicompartment micelles in which the emission of each segment can be controlled to produce colours throughout the visible spectrum. This represents a bottom-up synthetic route to objects analogous to nanoscale pixels, into which complex patterns may be written. Because of their small size and high density of encoded information, these findings could lead to the development of new materials for applications in, for example, biological diagnostics, miniaturized display technology and the preparation of encoded nanomaterials with high data density. While Nature routinely constructs complex biological structures with exquisite control, laboratory-based synthetic methods are only beginning to reach similar levels of precision in the creation of nanoscale architectures [1] , [2] , [3] , [4] , [5] , [6] , [7] . Advances in the preparation of soft matter nanostructures have recently made possible the preparation of a wide variety of objects with well-defined dimensions and hierarchies. In particular, emerging strategies based on the self-assembly of block copolymers (BCPs) have enabled the construction of objects with multiple domains physically segregated on the nanoscale, making it possible to design multifunctional structures with a high degree of spatial control [8] , [9] . Such methods have enabled the synthesis of functional nanoscale materials of increasing complexity, including photonic crystals [10] , dispersants [11] , polymer vesicles [12] , [13] , monochromatic barcodes [14] and therapeutic nanoconstructs [15] . In the face of increasing demand for miniaturization in areas such as optics, electronics and diagnostics, the fabrication of nanoscale luminescent materials with well-controlled sizes, shapes and emission colours has attracted intense interest. Quantum dots, for example, are a well-studied class of nanoscale objects whose emission colour can be controlled [16] , and recent reports have also described the preparation of nanorods [17] , microspheres [18] and nanocapsules [19] with tunable fluorescent emission. However, the preparation of nanoscopic objects that express multiple emission colours in a well-defined pattern has proven a challenge, in large part due to the difficulty in preventing energy transfer between emissive domains. Because of their small size and potentially high density of encoded information, such materials could have applications in multiplexed cellular diagnostics [20] and the invisible identification and tracking of valuable objects [21] , [22] . Crystallization-driven self-assembly (CDSA) of BCPs represents a useful emerging synthetic tool for the preparation of complex nanoscale architectures based on soft matter [23] . When crystalline-coil diblock copolymers are placed in a selective solvent for the coil block, crystallization of the core block drives the self-assembly of these BCPs to form low-curvature structures such as cylinders and platelets. In several cases, CDSA has been shown to be a ‘living’ process in the manner of a living covalent polymerization, as the ends of the resulting micelles remain active to the addition of further unimer (molecularly dissolved BCP) via epitaxial growth. For example, cylindrical structures of precise length and narrow length distributions can be created when unimers are added to short sonication-derived seed micelles, which act as initiation sites for CDSA [24] . Furthermore, block co-micelles with segmented structures are formed when different unimers are added sequentially to pre-existing seed initiators. CDSA phenomena have recently been reported for a wide variety of BCPs with different crystallizable core blocks [25] , [26] , [27] , and analogous processes have been used to form supramolecular heterojunctions from crystallizable hexabenzocoronene small molecules [28] . Using CDSA, we herein describe a versatile platform for the preparation of fluorescent nanoscale cylinders with fully tunable lengths and emission colours. Furthermore, using this method, the preparation of segmented cylindrical micelles is possible, where the colour of each segment can be precisely controlled. The preparation of non-centrosymmetric fluorescent multiblock micelles was also successfully achieved, providing a route to objects analogous to nanoscale pixels by low-cost solution processing. Finally, we demonstrate that these techniques may be used to fabricate encoded nanomaterials, giving fluorescent cylinders with the potential for extremely high data density. Synthesis of functional polymers To achieve our objectives, we targeted a block copolymer with a crystallizable polyferrocenyldimethylsilane (PFS) block [29] , [30] capable of CDSA such that a defined proportion of the coil block could be easily functionalized. The ability to control the loading of any functionality onto the corona is essential, as this can have a profound effect not only on the functional properties of the object but its self-assembly as well. We therefore synthesized block copolymers of the form PFS 62 - b -(PDMS 605 - r -PMVS 21 ), where PDMS=poly(dimethylsiloxane) and PMVS=poly(methylvinylsiloxane). Using this method, approximately 3% of randomly distributed vinyl groups along the coil block were introduced, which can serve as reactive sites for the introduction of more advanced functionality. These vinyl groups were then functionalized by photoinitiated hydrothiolation (thiol-ene ‘click’ reactions) [31] , [32] with either 2-mercaptoethanol or 2-mercaptoethylamine, providing primary hydroxyl or amino groups to which functional units may be attached. Fluorescent block copolymers capable of CDSA were then prepared by functionalization with a series of fluorophores based on a 4,4-difluoro-4-bora-3a,4a-diaza- s -indacene (BODIPY) core. BODIPY dyes have numerous advantages, such as large molar extinction coefficients, high quantum yields and relatively narrow absorption and emission bands, giving brightly emissive dyes which can be excited and detected independently of one another [33] . Furthermore, the emission colour of these dyes is highly tunable based on the functionalization of the BODIPY π-skeleton, with available colours from the blue to red regions of the visible spectrum. We thus prepared fluorescent polymers 1–3 that exhibit bright red, green and blue fluorescence, with emission maxima of 639, 516 and 456 nm in THF, respectively ( Fig. 1 ). 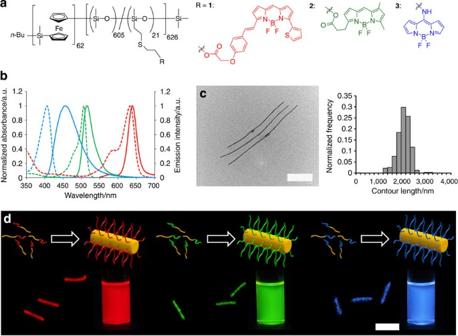Figure 1: Schematic of luminescent BCPs 1–3 and their self-assembly. (a) Structure of fluorescent BCPs1–3. (b) Normalized absorption (dashed) and emission (solid) spectra of unimers of1–3in THF, at dye concentrations of 10−5M. (c) Representative transmission electron microscopy (TEM) micrograph and corresponding contour length distribution of cylindrical micelles made from1–3. Scale bar, 500 nm. (d) Schematic representation of the self-assembly of1–3to form micelles, with corresponding confocal fluorescence micrographs and raw photographic images of micelle solutions under UV irradiation at 365 nm. Scale bar, 3 μm. Figure 1: Schematic of luminescent BCPs 1–3 and their self-assembly. ( a ) Structure of fluorescent BCPs 1–3 . ( b ) Normalized absorption (dashed) and emission (solid) spectra of unimers of 1–3 in THF, at dye concentrations of 10 −5 M. ( c ) Representative transmission electron microscopy (TEM) micrograph and corresponding contour length distribution of cylindrical micelles made from 1 – 3 . Scale bar, 500 nm. ( d ) Schematic representation of the self-assembly of 1–3 to form micelles, with corresponding confocal fluorescence micrographs and raw photographic images of micelle solutions under UV irradiation at 365 nm. Scale bar, 3 μm. Full size image Colour-tunable fluorescent micelles When solutions of 1–3 in THF (a good solvent for both blocks) are added to ethyl acetate (EtOAc), a selective solvent for PDMS and a poor solvent for PFS, these polymers readily self-assemble to form cylindrical micelles of core width ~10 nm via CDSA ( Supplementary Fig. 1 ). As we have shown previously, the lengths of these cylinders may be precisely controlled by first adding a sample of pre-formed crystallite seed micelle initiators (generated by sonication of longer cylinders) to serve as nucleation sites for self-assembly [24] . The resulting cylindrical nanostructures are highly fluorescent, with emission spectra approximately unchanged from those of the dissolved unimers in THF ( Fig. 1d ). Although important advances have recently been made in full-colour fluorescent reproduction on a molecular scale [34] , reproducing colours accurately using mixtures of dye molecules has long been problematic due to energy transfer, or cross-talk, between emitting materials. Physical separation of molecular emitters is typically required to achieve full-colour fluorescence, or dominant emission from the fluorophore with the lowest band gap is observed. Because of the difficulty in achieving such an arrangement, most strategies for obtaining full-colour emission have focused on precisely tuning the mixing ratios of dyes that experience some degree of energy transfer [35] , [36] , a process that is both time consuming and difficult to reproduce. We have therefore investigated an alternative approach involving the concurrent self-assembly of BCPs 1–3 into nanostructures doped with low concentrations of fluorescent dye, which offers an opportunity for facile reproduction of any colour within the gamut of the three primary colours ( Fig. 2 , Supplementary Fig. 2 , Supplementary Table 1 ). 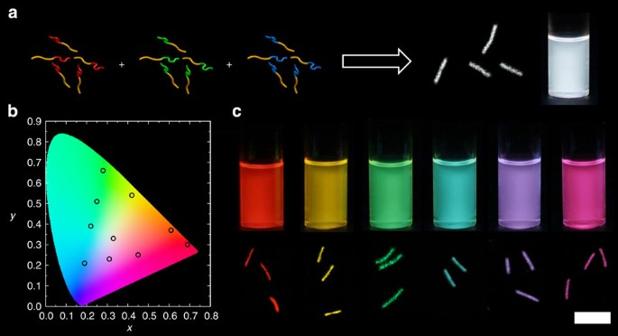Figure 2: Self-assembly of 1–3 into nanostructures of tunable colour. (a) Schematic representation showing the concurrent self-assembly of1–3to form micelles of tunable emission colour; white light-emitting micelles are shown as an example. (b) CIE 1931 chromaticity diagram showing the emission colour coordinates of the micelle solutions shown here. The coordinates of micelles made from only one of1,2or3represent the vertices of the triangle. (c) Raw photographic images of solutions of fluorescent micelles with tunable emission colour under UV irradiation at 365 nm, with corresponding LSCM images. Scale bar, 3 μm. Figure 2: Self-assembly of 1–3 into nanostructures of tunable colour. ( a ) Schematic representation showing the concurrent self-assembly of 1–3 to form micelles of tunable emission colour; white light-emitting micelles are shown as an example. ( b ) CIE 1931 chromaticity diagram showing the emission colour coordinates of the micelle solutions shown here. The coordinates of micelles made from only one of 1 , 2 or 3 represent the vertices of the triangle. ( c ) Raw photographic images of solutions of fluorescent micelles with tunable emission colour under UV irradiation at 365 nm, with corresponding LSCM images. Scale bar, 3 μm. Full size image The relative contributions of each fluorophore to the emission spectra of the resulting micelles were found to vary linearly with the composition of the BCP mixture, indicating that problematic energy transfer was negligible. Both the low loading of dye molecules in the corona and the tendency for the coronas to expand in a good solvent are expected to suppress short-range Dexter energy transfer processes, while Förster energy transfer is likely to be inefficient due to the poor overlap between the absorption and emission spectra of the three fluorophores used here. The fluorescence spectra that will result from any given mixture of 1–3 can thus be accurately predicted by additive colour theory (see Methods section), allowing for the synthesis of nanostructures with precisely defined emission colours. Furthermore, individual imaging of each colour by laser scanning confocal microscopy (LSCM) reveals the distribution of luminescence to be highly uniform, demonstrating that the overall colour is homogeneous along the length of the micelle ( Supplementary Fig. 3 ). Significantly, this method can be used to produce nanostructures exhibiting high quality white light emission, as micelles formed from a 1.03:0.75:1 ratio of polymers 1 : 2 : 3 exhibit luminescence with chromaticity coordinates of (0.33, 0.33). White light-emitting systems have long posed a challenge on the molecular scale and are of significant interest because of their potential uses in full-colour displays and lighting sources [35] , [36] , [37] . Finally, by mathematical prediction of the required polymer composition (see Methods section), we have prepared luminescent micelles with a chromaticity matching that of the D65 standard illuminant (0.31271, 0.32902), a common reference for the emission colour of daylight. Using the Commission internationale de l’éclairage (CIE) 1931 colour matching functions for a 2° standard observer, a 0.79:0.76:1 ratio of 1 : 2 : 3 is predicted to give this chromaticity. The preparation of such a sample gave micelles with an emission colour of (0.31, 0.33). Fluorescent multiblock micelles Because of the living nature of CDSA, additional unimers can be added to solutions of pre-formed micelles, forming block co-micelles with well-defined segments [38] . In the case of fluorescent polymers 1–3 , this provides a convenient method for the spatially defined nanosegregation of domains with variable fluorescent colour, which we refer to here as nanopixels. 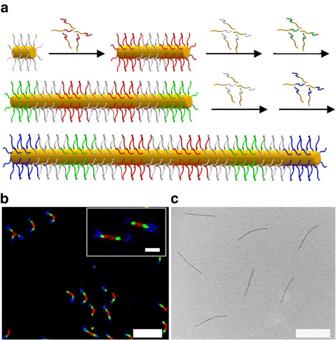Figure 3: Fluorescent 11-block micelles. (a) Schematic representation of fluorescent M(3)-b-M(PFS60-b-PDMS660)-b-M(2)-b-M(PFS60-b-PDMS660)-b-M(1)-b-M(PFS60-b-PDMS660)-b-M(1)-b-M(PFS60-b-PDMS660)-b-M(2)-b-M(PFS60-b-PDMS660)-b-M(3) 11-block co-micelles, where the prefix ‘M’ denotes that the block copolymer is incorporated into a micelle. PFS=yellow, PDMS=white, fluorescent coronas of1,2and3=red, green and blue, respectively. (b) LSCM image of fluorescent 11-block co-micelles. Scale bar, 5 μm. Inset scale bar, 1 μm. (c) Corresponding TEM micrograph. Scale bar, 3 μm. Figure 3 shows a sample of centrosymmetric 11-block co-micelles formed from the sequential addition of 1 , 2 and 3 to a solution of non-fluorescent seed initiators, with additional non-fluorescent spacers added between fluorescent segments to increase optical resolution ( Supplementary Fig. 4 ). These regions of colour are stable over a period of months with no detectable diffusion of luminescent polymers across the length of the micelles. Furthermore, the individual colours represented on the micelle are individually addressable due to the narrow absorption bands of the dyes ( Supplementary Fig. 5 ). It is thus possible to illuminate each colour individually, all three simultaneously, or any combination of two colours along the nanostructures. Although several reports have described the preparation of cylindrical nanostructures with segregated fluorescent regions [12] , [14] , [39] , this represents the first example of such structures where full control over the length, number and emission colour of the fluorescent regions can be achieved. Figure 3: Fluorescent 11-block micelles. ( a ) Schematic representation of fluorescent M( 3 )- b -M(PFS 60 - b -PDMS 660 )- b -M( 2 )- b -M(PFS 60 - b -PDMS 660 )- b -M( 1 )- b -M(PFS 60 - b -PDMS 660 )- b -M( 1 )- b -M(PFS 60 - b -PDMS 660 )- b -M( 2 )- b -M(PFS 60 - b -PDMS 660 )- b -M( 3 ) 11-block co-micelles, where the prefix ‘M’ denotes that the block copolymer is incorporated into a micelle. PFS=yellow, PDMS=white, fluorescent coronas of 1 , 2 and 3 =red, green and blue, respectively. ( b ) LSCM image of fluorescent 11-block co-micelles. Scale bar, 5 μm. Inset scale bar, 1 μm. ( c ) Corresponding TEM micrograph. Scale bar, 3 μm. Full size image Although a wide range of nanoscale morphologies are accessible through BCP self-assembly, relatively few examples exist of methods for the preparation of non-centrosymmetric, non-spherical structures [40] , [41] . However, non-centrosymmetric micelles can be accessed by CDSA using a unidirectional growth approach, by the generation of seed micelles capable of further epitaxial growth at one end only [42] . Addition of PFS 53 - b -PMVS 600 unimer to pre-formed PFS 60 - b -PDMS 660 micelles gives B-A-B triblock micelles of the form M(PFS 53 - b -PMVS 600 )- b -M(PFS 60 - b -PDMS 660 )- b -M(PFS 53 - b -PMVS 600 ) ( Supplementary Fig. 6 ). Addition of a radical photoinitiator and irradiation with UV light then results in the cross-linking of the PMVS coronas [43] , rendering these micelle blocks stable to the addition of a good solvent for PFS, PDMS and PMVS ( Supplementary Fig. 7 ). After dissolving the central, non-cross-linked micelle block by stirring the solution with 30% THF (v/v), non-centrosymmetric micelles could be obtained after dialysis back into pure EtOAc ( Supplementary Fig. 8 ). To this solution, unimers of 1–3 were then sequentially added, spaced out by small segments of non-fluorescent BCP. The result is a 7-block non-centrosymmetric cylindrical nanostructure that exhibits spatially segregated red, green and blue fluorescence, analogous to a nanoscale set of RGB pixels ( Fig. 4 , Supplementary Figs 9–10 ). 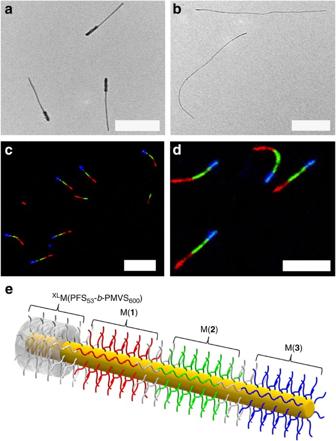Figure 4: Non-centrosymmetric RGB nanopixels. (a) TEM micrograph ofXLM(PFS53-b-PMVS600)-b-M(PFS60-b-PDMS660)-b-M(1) triblock co-micelles, formed after addition of1to a solution of non-centrosymmetricXLM(PFS53-b-PMVS600)-b-M(PFS60-b-PDMS660) micelles. ‘XL’ indicates that the block has been crosslinked. Scale bar, 500 nm. (b) TEM micrograph of 7-blockXLM(PFS53-b-PMVS600)-b-M(PFS60-b-PDMS660)-b-M(1)-b-M(PFS60-b-PDMS660)-b-M(2)-b-M(PFS60-b-PDMS660)-b-M(3) co-micelles. Scale bar, 2 μm. (c,d) LSCM micrographs of 7-block RGB nanopixels. Scale bar, 10 μm (c) 5 μm (d). (e) Schematic representation of 7-block RGB nanopixels. Figure 4: Non-centrosymmetric RGB nanopixels. ( a ) TEM micrograph of XL M(PFS 53 -b- PMVS 600 ) -b- M(PFS 60 -b- PDMS 660 ) -b- M( 1 ) triblock co-micelles, formed after addition of 1 to a solution of non-centrosymmetric XL M(PFS 53 -b- PMVS 600 ) -b- M(PFS 60 -b- PDMS 660 ) micelles. ‘XL’ indicates that the block has been crosslinked. Scale bar, 500 nm. ( b ) TEM micrograph of 7-block XL M(PFS 53 -b- PMVS 600 ) -b- M(PFS 60 -b- PDMS 660 ) -b- M( 1 ) -b- M(PFS 60 -b- PDMS 660 ) -b- M( 2 ) -b- M(PFS 60 -b- PDMS 660 ) -b- M( 3 ) co-micelles. Scale bar, 2 μm. ( c , d ) LSCM micrographs of 7-block RGB nanopixels. Scale bar, 10 μm ( c ) 5 μm ( d ). ( e ) Schematic representation of 7-block RGB nanopixels. Full size image The present system also provides a convenient method for the preparation of encoded nanomaterials, bearing a defined pattern with fluorescence as the output signal. Such materials are increasingly sought after as a method for invisibly identifying valuable objects or conveying sensitive information, and several examples of on/off nanoscale barcodes capable of binary encoding have been described [14] , [21] , [22] , [44] . Here, however, the ability to control the number of micelle blocks as well as fully tune the colour of each block allows for the preparation of nanomaterials with more complex patterns as well as vastly increased data density. For example, here we report micelles with 18 distinct, readily identifiable colours, as well as non-centrosymmetric structures with up to seven blocks. While many more colours can be prepared, with just this platform it is in principle possible to fabricate micelles with 18^7, or 6.1 × 10 8 combinations of fluorescent colour. This not only far exceeds the data density of binary encoding, but facilitates the encoding of nanostructures with more complex patterns as well. As a proof of concept, we demonstrate the preparation of luminescent pentablock co-micelles representing the colours of the flags of Canada, the United Kingdom and Ireland ( Fig. 5 ). These materials are indistinguishable by electron microscopy ( Fig. 5a–c ), but, when examined using confocal fluorescence microscopy, their encoded patterns are revealed ( Fig. 5d–f ). 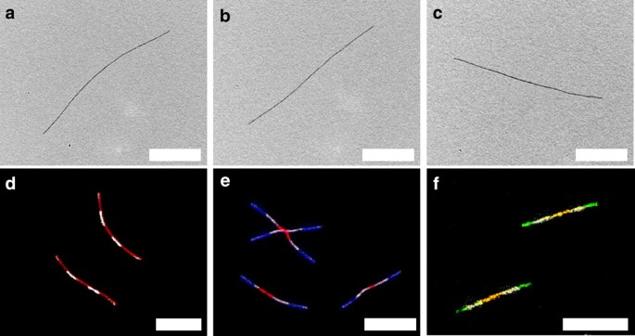Figure 5: Micelles with complex-encoded fluorescence. TEM micrographs and corresponding LSCM images of pentablock micelles with encoded colour patterns: (a,d) red-white-red-white-red fluorescent micelles, (b,e) blue-white-red-white-blue fluorescent micelles and (c,f) green-white-orange-white-green micelles. Scale bar, 2 μm (a–c), 5 μm (d–f). Figure 5: Micelles with complex-encoded fluorescence. TEM micrographs and corresponding LSCM images of pentablock micelles with encoded colour patterns: ( a , d ) red-white-red-white-red fluorescent micelles, ( b , e ) blue-white-red-white-blue fluorescent micelles and ( c , f ) green-white-orange-white-green micelles. Scale bar, 2 μm ( a – c ), 5 μm ( d–f ). Full size image In summary, using a series of fluorescent BCPs and the CDSA method we have prepared nanoscale pixels of fully tunable colour, whose emission characteristics can be precisely controlled. Such structures may find uses in the further miniaturization of imaging and diagnostics, including in biological systems where cylindrical probes have recently been shown to persist in circulation for far longer than spheres [45] . CDSA has also been used to construct monodisperse cylindrical multiblock nanostructures with distinct domains, each with its own persistent and tunable colour. Furthermore, we have used this method to prepare non-centrosymmetric, self-assembled RGB nanopixels. This technology can further be extended to hierarchical structures, whereby short arrays of axially aligned RGB micelles can be prepared using a platelet micelle as a template ( Supplementary Fig. 11 ). As the preparation of these multiblock micelles requires only the sequential addition of unimer, these processes may be easily automated for the high-throughput synthesis of nanostructures with complex encoded fluorescence. General experimental considerations Anionic polymerizations were carried out in an argon atmosphere glovebox. All other manipulations were carried out under an open atmosphere unless otherwise stated. PFS 60 -b- PDMS 660 , PFS 63 -b- PDMS 513 and PFS 53 -b- PMVS 600 were prepared by previously reported methods [46] . BODIPY 630/650 was purchased from Life Technologies Corporation; all other reagents were purchased from Sigma-Aldrich unless otherwise stated. Monomer purifications were performed under an atmosphere of purified N 2 . Hexamethylcyclotrisiloxane (D 3 ) was dissolved in pentane and stirred over CaH 2 for 48 h. Subsequently, the pentane was distilled off and the D 3 was consecutively sublimed under reduced pressure three times. Pentamethylvinylcyclotrisiloxane (VD 2 ) was prepared by literature methods [47] , [48] and distilled over CaH 2 . THF was distilled from Na/benzophenone immediately before use. 4,4-difluoro-5,7-dimethyl-4-bora-3a,4a-diaza-s-indacene-3-propionic acid (BODIPY-FL) [49] and 4,4-difluoro-4-bora-3a,4a-diaza-8-thiomethyl- s -indacene (8-thiomethylBODIPY) [50] were synthesized by previously reported methods. UV/Vis data were obtained on a Lambda 35 Spectrometer employing standard quartz cells with a path length of 1 cm. Fluorescence spectra were obtained on a Perkin–Elmer LS 45 fluorescence spectrometer using an excitation wavelength ( λ ex ) of 365 nm and are corrected for the sensitivity of the detector. CIE 1931 chromaticity coordinates were calculated against the CIE 1931 2° observer functions using standard methods [51] . Photoirradiation experiments were carried out with Pyrex-glass filtered emission from a 125 W medium-pressure mercury lamp (Photochemical Reactors Ltd.). An ethylene glycol/water bath in conjunction with a thermostat was used to maintain constant temperatures of 20 °C during the photoirradiation experiments. 1 H and 13 C NMR spectra were recorded using Jeol Eclipse 400 MHz or Varian VNMR 400 MHz spectrometers. Micelle photographs were taken using a Canon EOS 350D digital SLR camera and have not been digitally edited. Polymer characterization Gel permeation chromatography was carried out on diblock copolymers and aliquots of the first block using a Viscotek VE 2001 Triple-Detector Gel Permeation Chromatograph equipped with an automatic sampler, a pump, an injector, an inline degasser and a column oven operating at 30 °C (see Supplementary Fig. 12 ). The elution columns consist of styrene/divinyl benzene gels with pore sizes between 500 Å and 100,000 Å. Detection was conducted by means of a VE 3580 refractometer, a four-capillary differential viscometer, and 90° and low angle (7°) laser light ( λ 0 =670 nm) scattering detectors, VE 3210 & VE 270. THF (Fisher) was used as the eluent, with a flow rate of 1.0 ml min −1 . Samples were dissolved in the eluent (2 mg ml −1 ) and filtered with a Ministart SRP 15 filter (polytetrafluoroethylene membrane of 0.45 μm pore size) before analysis. The calibration was conducted using a PolyCAL polystyrene standard (PS115K) from Viscotek. Matrix-assisted laser desorption/ionization time of flight (MALDI-TOF) mass spectrometry measurements of polyferrocenyldimethylsilane (PFDMS) were performed using a Bruker Ultraflextreme running in the linear mode. Samples were prepared using a 1,8-dihydroxy-9,10-dihydroanthracen-9-one (dithranol) matrix (20 mg ml −1 in THF) and the polymer sample (2 mg ml −1 in THF), mixed in a 10:1 (v/v) ratio. Approximately 1 μl of the mixed solution was deposited onto a MALDI sample plate and allowed to dry in air. The molecular weights of the diblock copolymers were then determined by combining the molecular weight M n of the first block from MALDI-TOF measurements with the block ratio of the diblock copolymer obtained by integrating the 1 H NMR spectroscopic signal intensities of the respective blocks (see Supplementary Table 2 ). DSC analyses were performed on a TA Instruments Q100 coupled to a RCS90 refrigerated cooling system at a scanning rate of 10 °C min −1 . The DSC samples were placed in hermetic aluminum pans and were tared using a XT220A Precisa microbalance before analysis. Transmission electron microscopy Copper grids from Agar Scientific, mesh 400, were coated with a carbon film. Carbon coating was done using an Agar TEM Turbo Carbon Coater where carbon was sputtered onto mica sheets before deposition on the grids via flotation on water. The samples for electron microscopy were prepared by drop casting one drop ( ca. 10 μl) of the micelle colloidal solution onto a carbon-coated copper grid, which was then placed on a piece of filter paper to remove excess solvent. Bright field TEM micrographs were obtained on a JEOL1200EX II microscope operating at 120 kV and equipped with an SIS MegaViewIII digital camera. Images were analysed using the ImageJ software package developed at the US National Institute of Health. For the statistical length analysis, approximately 300–400 cylinders were carefully traced by hand to determine the contour length. Each TEM micrograph was analysed completely, that is, every cylindrical micelle in each image was counted to reduce subjectivity. Histograms of the length distribution were constructed. From this data, values of the standard deviation of the length distribution ‘sigma’ were determined. In addition, values of L n and L w of each sample were calculated as shown below ( L =length of object, N =number). Confocal fluorescence microscopy Confocal imaging was performed using a Leica SP5 system attached to a Leica DMI6000 inverted epifluorescence microscope with a × 63 (NA 1.4) oil immersion objective lens. Fluorophores from polymers 1 , 2 and 3 were excited using a HeNe laser operating at 594 nm, an argon laser operating at 488 nm and a UV diode laser operating at 405 nm, respectively. Confocal images were obtained using digital detectors with observation windows of 605–700 nm for 1 , 500–570 nm for 2 and 415–470 nm for 3 . The resulting outputs are obtained as digital false-colour images, which are colour-coded using the chromaticity of each micelle block under UV irradiation at 365 nm, as observed by fluorescence spectroscopy. For imaging of multiblock micelles, the output power of each laser was varied until the fluorescence of all blocks could be observed at approximately equal brightness. Micelle concentrations of 0.01 mg ml −1 in EtOAc were used for imaging experiments. Mathematics for accurate colour reproduction The tristimulus values X , Y and Z for a given emission spectrum Φ(λ) may be obtained by integration of the spectrum against the colour matching functions x (λ), y (λ) and z (λ), respectively, where x (λ), y (λ) and z (λ) represent the CIE 1931 colour matching functions for a 2° standard observer: The chromaticity of the spectrum of luminance Y is then given by the two parameters x and y , such that: For three emission sources with spectra Φ R (λ), Φ G (λ) and Φ B (λ), the tristimulus values for each spectrum are thus given by ( X R , Y R , Z R ), ( X G , Y G , Z G ) and ( X B , Y B , Z B ), respectively. For an emission spectrum Φ M (λ) obtained by mixing of Φ R (λ), Φ G (λ) and Φ B (λ) in a ratio of r:g:b , the tristimulus values ( X M , Y M , Z M ) will be given by: and the chromaticity values x M , y M defined as in equation 4. For a given set of chromaticity values x M , y M and luminance Y M , it follows that the tristimulus values X M and Z M may be obtained by: By combining equations 5 and 6, we find that for a desired chromaticity x M , y M with luminance Y M , the mixing ratio r:g:b of emission spectra Φ R (λ), Φ G (λ) and Φ B (λ) may be determined precisely via: Thus, the mixing ratio r:g:b can be obtained for arbitrary chromaticity coordinates x M , y M . Synthesis Polyferrocenylsilane 62 -b- [poly(dimethylsiloxane) 605 - r -poly(methylvinylsiloxane) 21 ] (PFS 62 -b- (PDMS 605 - r -PMVS 21 ): In a glove box under an argon atmosphere 1.6 M n -butyllithium (22 μl, 0.035 mmol) was added in one portion to a vigorously stirring solution of dimethylsila[1]ferrocenophane (0.500 g, 2.06 mmol) in dry THF (10 ml) in a greaseless Schlenk flask. The reaction mixture was stirred for 1.5 h over which time the colour changed from red to orange. An aliquot (0.2 ml) for later analysis was removed, diluted with THF (1 ml) and quenched with 3,5-di- tert -butyl-4-hydroxytoluene. To the remaining reaction mixture, a solution of 1,3,3,5,5-pentamethyl-1-vinylcyclotrisiloxane (0.145 g, 0.62 mmol) and 1,1,3,3,5,5-hexamethylcyclotrisiloxane (1.39 g, 6.2 mmol) in dry THF (2 ml) was added in one portion. After 2 h, the flask was removed from the glove box, set up under a nitrogen atmosphere and the reaction quenched with a few drops of chlorotrimethylsilane. The product was precipitated once in methanol with 10% triethylamine and twice more in methanol. To remove the homopolymer, the crude product was dissolved in a minimum amount of THF and ethyl acetate was added with stirring until the solution became cloudy. The suspension was centrifuged at 6,000 r.p.m. for 15 min and the supernatant concentrated in vacuo , precipitated in methanol and dried in vacuo at 40 °C to afford the pure block copolymer (1.467 g, 73%) as an orange solid. δ H (500 MHz; CD 2 Cl 2 ) 6.07–5.90 (m, 42H, CHC H 2 ), 5.85–5.76 (m, 21H, SiC H CH 2 ), 4.23 (s, 248H, Cp H ), 4.02 (s, 248H, Cp H ), 0.47 (s, 372H, FcSi(C H 3 ) 2 ), 0.15 (s, 63H, Si(CHCH 2 )C H 3 ), 0.08 (s, 3630H, Si(CH 3 ) 2 ) p.p.m. ; δ C (100 MHz; CD 2 Cl 2 ) 73.7 (Cp C ), 72.2 (Cp C Si), 71.8 (Cp C ), 1.3 (OSi( C H 3 ) 2 ), −0.8 (SiCH 3 ) 2 p.p.m. ; δ Si (99 MHz, CD 2 Cl 2 ) −6.9, −21.8 p.p.m. ; PDI=1.06. Hydrothiolation of PFS 62 -b- (PDMS 605 -r-PMVS 21 ) with 2-hydroxyethanethiol (4) : To a solution of PFS 62 -b- (PDMS 605 -r-PMVS 21 ) (205 mg, 3.2 × 10 −3 mmol, 0.070 mmol vinyl groups) in dry THF (3 ml) was added 2-mercaptoethanol (18 μl, 20 mg, 0.21 mmol, 3 equiv.) and the photo-initiator 2,2-dimethoxy-2-phenylacetophenone (2 mg, 7.8 × 10 −3 mmol). The orange solution was sealed under an argon atmosphere and irradiated 3 cm away from a mercury lamp for 1 h. The mixture was then precipitated three times into methanol and dried in vacuo at 40 °C to afford the pure block copolymer (202 mg, 96%). 1 H NMR analysis showed quantitative functionalization of the siloxane vinyl groups with 2-thioethanol. δ H (400 MHz; CD 2 Cl 2 ) 4.23 (s, 248H, Cp H ), 4.02 (s, 248H, Cp H ), 3.66 (m, 42H, C H 2 OH), 2.70 ( t , J=6.1Hz, 42H, SC H 2 ), 2.58 (m, 42H, SC H 2 ), 0.87 (m, 42H, SiC H 2 CH 2 S), 0.47 (s, 372H, FcSi(C H 3 ) 2 ), 0.08 (s, 3693H, Si(C H 3 )) p.p.m. ; δ C (100 MHz; CD 2 Cl 2 ) 73.7 (Cp C ), 72.2 (Cp C Si), 71.8 (Cp C ), 1.3 (OSi( C H 3 ) 2 ), −0.8 (SiCH 3 ) 2 p.p.m. ; δ Si (99 MHz, CD 2 Cl 2 ) −6.9, −21.8 p.p.m. ; PDI=1.17. Hydrothiolation of PFS 62 -b- (PDMS 605 -r-PMVS 21 ) with 2-aminoethanethiol (5) : To a solution of PFS 62 -b- (PDMS 605 -r-PMVS 21 ) (200 mg, 3.1 × 10 −3 mmol, 0.068 mmol vinyl groups) in dry THF (3 ml) was added 2-mercaptoethylamine hydrochloride (77 mg, 0.68 mmol, 10 equiv.) and the photo-initiator 2,2-dimethoxy-2-phenylacetophenone (2 mg, 7.8 × 10 −3 mmol). The orange solution was sealed under an argon atmosphere and irradiated 3 cm away from a mercury lamp for 4 h. The mixture was then precipitated three times into methanol and dried in vacuo at 40 °C to afford the pure block copolymer (163 mg, 80%). 1 H NMR analysis showed quantitative functionalization of the siloxane vinyl groups with 2-aminoethanethiol. δ H (400 MHz; CD 2 Cl 2 ) 4.23 (s, 248H, Cp H ), 4.02 (s, 248H, Cp H ), 2.80 ( t , J=6.4 Hz, 42H, SC H 2 ), 2.60–2.53 (m, 84H, SC H 2 +C H 2 NH 2 ), 0.87 (m, 42H, SiC H 2 CH 2 S), 0.48 (s, 372H, FcSi(C H 3 ) 2 ), 0.08 (s, 3693H, Si(C H 3 )) p.p.m. ; δ C (100 MHz; CD 2 Cl 2 ) 73.7 (Cp C ), 72.2 (Cp C Si), 71.8 (Cp C ), 1.3 (OSi( C H 3 ) 2 ), −0.8 (SiCH 3 ) 2 p.p.m. ; δ Si (99 MHz, CD 2 Cl 2 ) −6.9, −21.8 p.p.m. ; PDI=1.82. Synthesis of PFS 62 -b- (PDMS 605 -r-PMVS 21 ) functionalized with BODIPY-630/650 dye (1) : To a 7 ml screw-cap vial with stir bar was added hydroxyl-functionalized PFS 62 -b- (PDMS 605 -r-PMVS 21 ) 4 (39 mg, 6.0 × 10 −4 mmol, 0.012 mmol hydroxyl groups), dicyclohexylcarbodiimide (4.8 mg, 0.033 mmol, 1.4 equiv. ), 4-dimethylaminopyridine (0.56 mg, 0.007 mmol, 0.3 equiv. ), 6-((4,4-difluoro-5-(2-thienyl)-4-bora-3a,4a-diaza- s -indacene-3-yl)styryloxy)acetic acid (BODIPY 630/650, 8 mg, 0.018 mmol, 1.4 equiv.) and 4 ml dry dichloromethane. The reaction was stirred under an argon atmosphere at room temperature for 72 h, then precipitated five times into methanol and dried in vacuo at 40 °C to afford the pure block copolymer (14 mg, 32%). 1 H NMR analysis showed 10% functionalization of the hydroxyl functional groups with BODIPY-630/650 dye, with 90% hydroxyl groups remaining. δ H (400 MHz; CD 2 Cl 2 ) 8.15 (d, J=3.7 Hz, 2H, thienyl Ar- H ), 7.61 (d, J=8.2 Hz, 4H, -C 6 H 4 -), 7.58 (d, J=16.5 Hz, 2H, =C H ), 7.52 (d, J=4.6 Hz, 2H, thienyl Ar- H ), 7.39 (d, J=16.5 Hz, 2H, =C H ), 7.21 (t, J=4.4 Hz, 2H, thienyl Ar- H ), 7.13 (s, 1H, C H between pyrroles), 7.11 (d, J=4.3 Hz, pyrrole Ar- H ), 7.04 (d, J=4.0 Hz, 2H, pyrrole Ar- H ) 7.00 (d, J=4.0 Hz, pyrrole Ar- H ), 6.95 (d, J=8.2 Hz, 4H, -C 6 H 4 -), 6.82 (d, J=4.3 Hz, 2H, pyrrole Ar- H ), 4.69 (s, 4H, C H 2 ), 4.34 (t, J=7.2 Hz, C H 2 OR), 4.23 (s, 248H, Cp H ), 4.02 (s, 248H, Cp H ), 3.67 (m, 38H, C H2 OH), 2.70 (t, J=6.0 Hz, 42H, SiCH 2 C H 2 S), 2.64 (m, 4H, SC H 2 CH 2 OR), 2.59 (m, 38H, SC H 2 CH 2 OH), 0.88 (m, 42H, SiC H 2 CH 2 S), 0.48 (s, 372H, FcSi(C H 3 ) 2 ), 0.08 (s, 3693H, Si(C H 3 )) p.p.m. ; δ C (100 MHz; CD 2 Cl 2 ) 73.7 (Cp C ), 72.2 (Cp C Si), 71.8 (Cp C ), 1.3 (OSi( C H 3 ) 2 ), −0.8 (SiCH 3 ) 2 p.p.m. ; δ Si (99 MHz, CD 2 Cl 2 ) −6.9, −21.8 p.p.m. ; PDI=1.60. Synthesis of PFS 62 -b- (PDMS 605 -r-PMVS 21 ) functionalized with BODIPY-FL dye (2) : To a 20 ml screw-cap vial flask with stir bar was added hydroxyl-functionalized PFS 62 -b- (PDMS 605 -r-PMVS 21 ) 4 (86 mg, 1.310 −3 mmol, 0.029 mmol hydroxyl groups), dicyclohexylcarbodiimide (17.6 mg, 0.087 mmol, 3 equiv. ), 4-dimethylaminopyridine (2.1 mg, 0.017 mmol, 0.6 equiv. ), 4,4-difluoro-5,7-dimethyl-4-bora-3a,4a-diaza- s -indacene-3-propionic acid (BODIPY-FL, 25.4 mg, 0.087 mmol, 3 equiv.) and 6 ml dry dichloromethane. The reaction was stirred under an argon atmosphere at room temperature for 72 h, then precipitated three times into methanol and dried in vacuo at 40 °C to afford the pure block copolymer (93 mg, 99%). 1 H NMR analysis showed quantitative functionalization of the hydroxyl functional groups with BODIPY-FL dye. δ H (400 MHz; CD 2 Cl 2 ) 7.13 (s, 21H, Ar H ), 6.90 (s, 21H, Ar H ), 6.27 (s, 21H, Ar H ), 6.15 (s, 21H, Ar H ), 4.23 (s, 248H, Cp H ), 4.21 (t, J=7.3 Hz, 42H, C H 2 OR), 4.02 (s, 248H, Cp H ), 3.22 (t, J=7.3 Hz, 42H, SC H 2 ), 2.77-2.70 (m, 84H, C(O)C H 2 +SC H 2 ), 2.62 (m, 42H, SC H 2 ), 2.53 (s, 63H, ArC H 3 ), 2.25 (s, 63H, ArC H 3 ), 0.88 (42H, SiC H 2 CH 2 S), 0.47 (s, 372H, FcSi(C H 3 ) 2 ), 0.08 (s, 3693H, Si(C H 3 )) p.p.m. ; δ C (100 MHz; CD 2 Cl 2 ) 73.7 (Cp C ), 72.2 (Cp C Si), 71.8 (Cp C ), 1.3 (OSi( C H 3 ) 2 ), −0.8 (SiCH 3 ) 2 p.p.m. ; δ Si (99 MHz, CD 2 Cl 2 ) −6.9, −21.8 p.p.m. ; PDI=1.21. Synthesis of PFS 62 -b- (PDMS 605 -r-PMVS 21 ) functionalized with 8-aminoethyl BODIPY dye (3) : To a 20 ml screw-cap vial with stir bar was added amine-functionalized PFS 62 -b- (PDMS 605 -r-PMVS 21 ) 5 (79 mg, 1.2 × 10 −3 mmol, 0.026 mmol amine groups), 8-methylthio-4,4-difluoro-4-bora-3 a,4 a-diaza-s-indacene (8-methylthio-BODIPY, 30 mg, 0.125 mmol, 5 equiv.) and 6 ml dichloromethane. The mixture was stirred under an atmosphere of air for 72 h then precipitated three times into methanol and dried in vacuo at 40 °C to afford the pure block copolymer (68 mg, 81%). 1 H NMR analysis showed quantitative functionalization of the amine functional groups with BODIPY dye. δ H (400 MHz; CD 2 Cl 2 ) 7.53–7.34 (m, br, 42H, Ar- H ), 7.25–6.99 (m, br, 42H, Ar- H ), 6.62–6.36 (m, br, 42H, Ar- H ), 4.23 (s, 248H, Cp H ), 4.02 (s, 248H, Cp H ), 3.95–3.76 (m, br, 42H, C H 2 NH), 3.07–2.87 (m, 42H, C H 2 S), 2.69–2.57 (m, 42H, C H 2 S), 0.97–0.80 (m, 42H, SiC H 2 CH 2 S), 0.48 (s, 372H, FcSi(C H 3 ) 2 ), 0.08 (s, 3693H, Si(C H 3 )) p.p.m. ; δ C (100 MHz; CD 2 Cl 2 ) 73.7 (Cp C ), 72.2 (CpCSi), 71.8 (Cp C ), 1.3 (OSi( C H 3 ) 2 ), −0.8 (Si C H 3 ) 2 p.p.m. ; δ Si (99 MHz, CD 2 Cl 2 ) −6.9, −21.8 p.p.m. ; PDI=1.38. Full Methods are available in the Supplementary Information . How to cite this article: Hudson, Z. M. et al . Colour-tunable fluorescent multiblock micelles. Nat. Commun. 5:3372 doi: 10.1038/ncomms4372 (2014).